Vortex flows impart chirality-specific lift forces Recent reports that macroscopic vortex flows can discriminate between chiral molecules or their assemblies sparked considerable scientific interest both for their implications to separations technologies and for their relevance to the origins of biological homochirality. However, these earlier results are inconclusive due to questions arising from instrumental artifacts and/or insufficient experimental control. After a decade of controversy, the question remains unresolved—how do vortex flows interact with different stereoisomers? Here, we implement a model experimental system to show that chiral objects in a Taylor–Couette cell experience a chirality-specific lift force. This force is directed parallel to the shear plane in contrast to previous studies in which helices, bacteria and chiral cubes experience chirality-specific forces perpendicular to the shear plane. We present a quantitative hydrodynamic model that explains how chirality-specific motions arise in non-linear shear flows through the interplay between the shear-induced rotation of the particle and its orbital translation. The scaling laws derived here suggest that rotating flows can be used to achieve chiral separation at the micro- and nanoscales. The idea that fluid flows can discriminate between chiral objects of opposite handedness was initially proposed by Howard et al. [1] and has since been examined theoretically in considerable detail [2] , [3] , [4] , [5] , [6] , [7] , [8] , [9] , [10] . Achieving separation of enantiomers [11] , [12] without the use of a chiral stationary phase—the most costly component in the separation process—would revolutionize the pharmaceutical industry. Surprisingly, however, there is still no agreement as to the magnitudes or even directions of forces affecting chiral objects in fluid flows [7] , [8] , [13] . Although several experimental studies report chirality-specific flow effects—on scales from molecular (porphyrin aggregation during rotary evaporation) [14] , [15] , through microscopic (helical bacteria [4] and particles [16] ), to macroscopic [13] , [17] , [18] —they remain largely phenomenological. Part of the problem is the possibly ambiguous interpretation of data [19] , [20] , [21] (for example, from circular dichroism) and the experimental design in which vortex flows are implemented with imprecise systems such as rotary evaporators or magnetic stirrers [22] , for which the flow structure on different length scales is largely unknown. In this study, we use the well-controlled flow generated in a Couette cell containing macroscopic chiral particles (confined to the liquid/air interface) to clarify and explain the chirality-selective motions of solid objects in non-linear shear flows. Importantly, by confining the motion of the particles to a two-dimensional (2D) interface, we are able to capture the detailed rotational and translational motion of the particles in time—not just their average drifting motion as in previous studies [4] , [16] , [18] . Such detailed experimental data allow for quantitative comparisons with predictions of the hydrodynamic model that we develop. Building on these experimental results, we develop quantitative scaling laws that describe how in-plane chiral-selective motions depend on the size and shape of the particle and on the geometry of the non-linear flow field. These scaling laws predict that rotating flows can provide physical means of separating chiral objects at the micro- and nanoscales. Experimental design Our experiments are performed in a custom-machined Couette cell ( Fig. 1a,b ) with the radius of the stationary inner cylinder R i =25.4±0.01 mm and that of the rotating outer cylinder R o =55.9±0.01 mm. The cylinders are aligned coaxially with variations in the gap width, G = R o − R i , <0.5 mm. The cell is partially filled with paraffin oil (dynamic viscosity, η =0.17±0.06 Pa·s; density, ρ =0.86±0.03 g ml −1 ) and in each experiment, a single millimetre-sized particle (7.70 × 2.46 × 0.20 mm, fabricated in SU-8 by photolithography; density 1.19 g ml −1 ) is placed onto the oil/air interface such that it is fully immersed in the oil save for its top face ( Fig. 1c ). The particles are s -shaped (D 2 h symmetry) such that when placed onto the interface, they have two non-superimposable—that is, chiral—orientations, which we denote ‘R’ and ‘S’ ( Fig. 1b ) by analogy to chemical convention. A shear flow is generated in the cell by rotating the outer cylinder (a configuration for which Taylor instabilities cannot occur) at an angular frequency ω cell =1–3 rad s −1 . For the typical particle dimensions and velocity, the particle Reynolds number is Re = ρLR o ω cell / η ~1 where L ≈4 mm is a characteristic linear dimension of the particle. 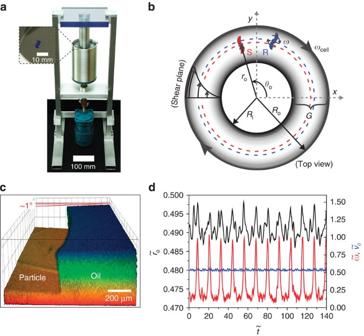Figure 1: Experimental arrangement. (a) Optical image of the Couette cell with a millimetre-sized chiral particle placed at the oil/air interface. (b) Top-view scheme of the system with an inner cylinder stationary and an outer cylinder rotating—here, in the CW direction—at an angular velocityωcell. Two chiral particles (denoted R and S) are illustrated; these particles revolve around the cell with linear velocityvθand also rotate around their centres with an angular velocityω. The shear plane is indicated by the curved arrows. (c) Three-dimensional confocal microscopy of a chiral particle floating stationary on top of paraffin oil (containing 1 μM diketopyrrolopyrrole to make the oil fluorescent). The particle is not fluorescent and therefore appears as a void space on the left of the image. No significant meniscus was observed; however, as the particle is slightly denser than the fluid, the interface slopes downward at ~1° near the particle edge (seeSupplementary Note 1). The grid size is 50 × 50 μm. (d) Typical experimental data showing the radial position(black), linear velocity(blue), and angular velocity(red) of an S particle as a function of time(after the particle has reached a stable orbit); here, the cell velocity isωcell=3.02±0.13 rad s−1. Figure 1: Experimental arrangement. ( a ) Optical image of the Couette cell with a millimetre-sized chiral particle placed at the oil/air interface. ( b ) Top-view scheme of the system with an inner cylinder stationary and an outer cylinder rotating—here, in the CW direction—at an angular velocity ω cell . Two chiral particles (denoted R and S) are illustrated; these particles revolve around the cell with linear velocity v θ and also rotate around their centres with an angular velocity ω . The shear plane is indicated by the curved arrows. ( c ) Three-dimensional confocal microscopy of a chiral particle floating stationary on top of paraffin oil (containing 1 μM diketopyrrolopyrrole to make the oil fluorescent). The particle is not fluorescent and therefore appears as a void space on the left of the image. No significant meniscus was observed; however, as the particle is slightly denser than the fluid, the interface slopes downward at ~1° near the particle edge (see Supplementary Note 1 ). The grid size is 50 × 50 μm. ( d ) Typical experimental data showing the radial position (black), linear velocity (blue), and angular velocity (red) of an S particle as a function of time (after the particle has reached a stable orbit); here, the cell velocity is ω cell =3.02±0.13 rad s −1 . Full size image Dynamics of chiral particles As the circular flow in the cell is established, the particles evolve within ~ 30 min to stable orbits. Importantly, the mean radii of these orbits depends on the particles’ chirality (R,S) but not on the initial particle position. All particle trajectories are recorded and analysed using house-written ImageJ and MATLAB scripts. The output of these scripts contain the linear velocity v θ of the particle in the θ -direction, the angular velocity ω of the particle about its centre, and the radial position r o of the particle centre measured from the axis of the Couette cell ( Fig. 1d ). Both R and S chiral particles revolve around the cell at a nearly constant speed v θ with variations of only ~3% about the mean ( Fig. 1d , blue line). On the other hand, the R and S particles exhibit large periodic variations in their angular velocities ω ( Fig. 1d , red line)—the so-called Jeffery orbits [23] characteristic of elongated particles in shear flows. The key experimental results of the present study are illustrated in Fig. 2a for R and S particles subject to clockwise (CW) and counter-clockwise (CCW) directions of cell rotation. For CW rotation, the mean radius of the orbit traced by the R particles is always greater than that of the S particles in the same flow, . In contrast, in a CCW flow, the opposite is true and . Moreover, and , which means that when the flow is reversed (from CW to CCW or from CCW to CW), the orbit of the R particle becomes that of S and vice versa. These results explicitly eliminate any influence of particle shape imperfections, centrifugal forces and capillarity on relative motions of R and S particles. The orbit radii change when only the flow is reversed and the particles are not manipulated in any way. Additional evidence that capillary effects are negligible comes from confocal microscopy imaging ( Fig. 1c ), which shows no appreciable meniscus between the immersed particle and the surrounding fluid (see also Supplementary Note 1 ). Furthermore, the above results indicate that the system can be treated as 2D whereby a hypothetical rotation of the Couette cell by 180 degrees around a horizontal axis ( Fig. 2b ) acts to reverse the apparent chirality of the particles and the direction of flow (for example, R→S and CW→CCW in Fig. 2b ) but does not alter the particle orbits. These symmetries require that and as observed in experiments. 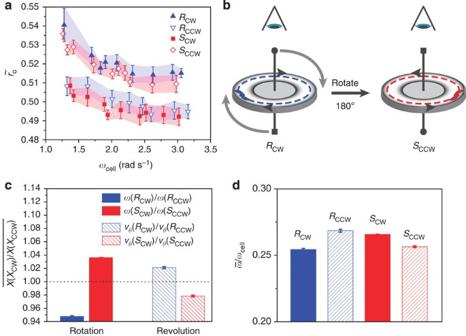Figure 2: Chirality effects in a vortex flow. (a) The mean orbit radiiobserved in experiments depends on the chirality of the particles and on the direction of flow (solid markers=CW cell rotation; open markers=CCW rotation). For all cell velocitiesωcell,and. Upon ‘flow reversal’ (without any manipulation of particles),and. Error bars correspond to standard deviations in, which are based on at least 10 independent experiments (12,500 data points per run recorded) for each value ofωcell(note: four particles of each type were tested). (b) Scheme illustrating why the behaviour of a chiral particle in a CW flow is expected to be equivalent to its ‘mirror image’ in a CCW flow. Rotation of the entire system by 180° about a horizontal axis (denoted by grey arrows) changes the particle chirality and the flow direction (with respect to an observer looking down the vertical axis as denoted by the eye cartoon) while the orbit radius remains unchanged. These symmetry arguments are in agreement with the experimental observations ina. (c) When the direction of flow reverses from CW to CCW, the linear and angular velocities,ωandvθ, also change as illustrated by the bar graph showing the ratios of the particle velocities for CW and CCW flows averaged over all experiments. Error bars represent s.d. based on at least 200 experiments for each bar. (d) The average angular velocity of the particlesis consistently smaller than that of the Couette cellωcell. Error bars represent s.d. based on at least 200 experiments for each bar. Figure 2: Chirality effects in a vortex flow. ( a ) The mean orbit radii observed in experiments depends on the chirality of the particles and on the direction of flow (solid markers=CW cell rotation; open markers=CCW rotation). For all cell velocities ω cell , and . Upon ‘flow reversal’ (without any manipulation of particles), and . Error bars correspond to standard deviations in , which are based on at least 10 independent experiments (12,500 data points per run recorded) for each value of ω cell (note: four particles of each type were tested). ( b ) Scheme illustrating why the behaviour of a chiral particle in a CW flow is expected to be equivalent to its ‘mirror image’ in a CCW flow. Rotation of the entire system by 180° about a horizontal axis (denoted by grey arrows) changes the particle chirality and the flow direction (with respect to an observer looking down the vertical axis as denoted by the eye cartoon) while the orbit radius remains unchanged. These symmetry arguments are in agreement with the experimental observations in a . ( c ) When the direction of flow reverses from CW to CCW, the linear and angular velocities, ω and v θ , also change as illustrated by the bar graph showing the ratios of the particle velocities for CW and CCW flows averaged over all experiments. Error bars represent s.d. based on at least 200 experiments for each bar. ( d ) The average angular velocity of the particles is consistently smaller than that of the Couette cell ω cell . Error bars represent s.d. based on at least 200 experiments for each bar. Full size image As expected for Taylor–Couette flow, in which flow velocity increases with radial position, particles revolving around larger orbits have higher velocities v θ —that is, (hatched bars in Fig. 2c ). At the same time, the average angular velocity of a particle decreases with increasing radial position—that is, (solid bars in Fig. 2c,d )—because depends linearly on the shear rate (ref. 23 ), which decreases with increasing r . Importantly, for achiral particles (disks or ellipsoids), no difference is observed in any of the measured variables ( Supplementary Fig. 1 ). Taken together, the above results indicate that the differences in the orbits of the R and S particles are due to their chirality. Because stable orbits correspond to the loci where all radial forces on the particles are balanced, we conclude that the R and S particles experience a lift force that is parallel to the shear plane (unlike in refs 2 , 4 , 7 , 18 ) and whose direction depends on the chirality of the object with respect to the flow. Hydrodynamic model of chirality-specific motions To gain further insight into the origin of this chiral lift, we consider the motion of a single rigid particle moving in the Taylor–Couette flow where e θ is the unit vector in the azimuthal direction. The particle is approximated by a collection of N small spheres of radius a that move together as a single object with linear velocity U and angular velocity ω . We first consider the limit of small Reynolds numbers ( Re ≪ 1) in which fluid inertia is negligible and the hydrodynamic force on sphere α can be approximated as where is the grand resistance tensor (see Methods), u ( r β ) is the flow velocity at the centre of sphere β, and v β =d r β /d t is the velocity of sphere β. Physically, this force originates from the motion of the sphere relative to that of the fluid and from hydrodynamic interactions with other spheres that make up the composite particle. The rigid body motion of the particle implies that the velocity of sphere β is related to that of the particle as v β = U + ω × R β where R β denotes the position of sphere β relative to the moving particle origin O (that is, R β = r β − r o ). To maintain the relative distances between the spheres, the hydrodynamic forces are exactly balanced by intraparticle forces between the spheres such that the net force F H and torque T H on the particle are identically zero Together with the kinematic conditions for rigid body motion, Equations (2) and (3) govern the dynamics of the particle position r o and its angular orientation (see Methods for details). This model is similar to that of Hänggi [6] and co-workers but includes hydrodynamic interactions between the spheres, which we found to have a significant impact on the magnitude of the chiral lift force and its scaling with particle size ( Supplementary Fig. 3 ). Numerical integration of the above equations provides several insights into the experimental observations ( Fig. 3 ). First, the linear velocity of the particle is roughly constant and equal to that of the fluid evaluated at the particle’s centre, v θ ≈ u θ ( r o ) (compare Figs 1d and 3b ). The angular velocity of the particle oscillates in time with a period equal to that of the particle’s rotation ( Fig. 3b ); the period of these Jeffery orbits is well approximated as where χ =3.1 is the aspect ratio of the particles and is the shear rate. Despite the simplifications involved, the hydrodynamic model predicts the particle rotation period in quantitative agreement with experiment—for example, for ω cell =3 rad s −1 , T =7.9 s in experiment as compared with T =7.2 s in the model using no tunable parameters. 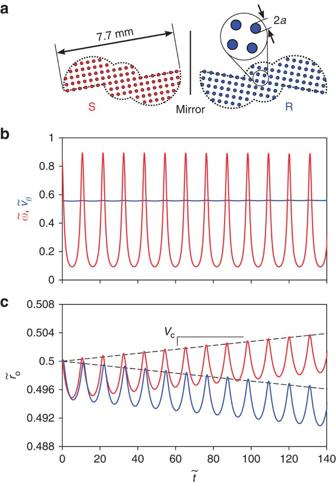Figure 3: Modelling of particle dynamics in Taylor–Couette flow. (a) Chiral particles (R and S) like those used in experiment are comprised ofN=91 spheres of radiusa=0.1 mm corresponding to the particle thickness; the spacing between neighbouring spheres is 4a. The characteristic linear dimension of the particle (assumed equal to the square root of its area) isL=4 mm; the dimensionless chiral factor isκ=1.9; and the aspect ratio isχ=3.1 (see Methods). (b) Numerical solution of the linear velocityand the angular velocityof an S particle moving in a CCW flow as a function of time. (c) The radial position of the particle’s centreoscillates in time with a steady drift velocityvcwhose direction depends on the chirality of the particle. Figure 3: Modelling of particle dynamics in Taylor–Couette flow. ( a ) Chiral particles (R and S) like those used in experiment are comprised of N =91 spheres of radius a =0.1 mm corresponding to the particle thickness; the spacing between neighbouring spheres is 4 a . The characteristic linear dimension of the particle (assumed equal to the square root of its area) is L =4 mm; the dimensionless chiral factor is κ =1.9; and the aspect ratio is χ =3.1 (see Methods). ( b ) Numerical solution of the linear velocity and the angular velocity of an S particle moving in a CCW flow as a function of time . ( c ) The radial position of the particle’s centre oscillates in time with a steady drift velocity v c whose direction depends on the chirality of the particle. Full size image Importantly, the radial position of the particle also oscillates in time but with a steady drifting motion that depends on both the chirality of the particle and the direction of the flow. For CCW rotation of the outer cylinder ( ω cell >0), S particles drift away from the origin while R particles drift toward the origin in agreement with experimental observations; the opposite behaviour is observed for CW rotation. A detailed scaling analysis of the hydrodynamic model reveals that the chiral drift velocity v c is well approximated as v c ≈ κaL / Tr o , where κ is a dimensionless ‘chiral factor’ that characterizes the direction and magnitude of the chiral drift and depends only on the shape of the particle (see Methods); for the model particles used in the simulations, κ (S)=− κ (R)=1.9. In the absence of inertial effects or hydrodynamic interactions with the walls of the Couette cell, chiral particles drift monotonically towards or away from the centre of the rotating flow. To understand the formation of the stable orbits observed in experiment, it is necessary to consider the role of fluid inertia, which acts to centre the particle within the gap separating the concentric cylinders. Near the midline position, , the inertial lift velocity v i has been calculated previously [24] for spherical particles to be v i ( r )≈( r m − r )/ τ , where is a characteristic time for the particle to relax to the steady-state orbit r m . For chiral particles, the chiral drift velocity is expected to perturb the orbit of the particle away from r m ; the resulting steady-state orbit r ss corresponds to that at which the chiral drift velocity balances the restoring lift velocity, v c ( r ss )≈ v i ( r ss ). Using the above estimates, the difference in the steady-state orbits between R and S particles is estimated as Δ r ss ≈ τv c ( r m )~1 mm and the relaxation time as τ ~10 min, both of which are in quantitative agreement with experiment. Interestingly, this mechanism also predicts that larger separations between chiral particles can be achieved at lower Reynolds numbers. This prediction is supported by experiments that show that the chiral separation Δ r ss increases from 2.3 to 3.0 mm as the rotation speed is reduced by a factor of two ( Fig. 2a ). Physical origins of chirality-specfic motions Analysis of the hydrodynamic model reveals that chiral drift parallel to the shear plane occurs through a previously unreported mechanism requiring the presence of non-linear flow fields (that is, ∇ ∇ u ≠0). In general, the hydrodynamic force/torque on a rigid particle depends both on its linear/angular velocity and on the fluid velocity u as where is the particle resistance tensor, are n th order tensors that depend on the shape and size of the particle, and the velocity gradients are evaluated at the particle origin O (see Methods) [25] , [26] , [27] , [28] . To first approximation, a force and torque-free particle moves at the local fluid velocity ( u o ) and rotates at a rate equal to one-half the local fluid vorticity (½ ∇ × u o ). Deviations of the particle’s translational and rotational velocity from that of the fluid are caused by straining flows which are incompatible with the rigid body motion of the particle. To describe these effects, it is most common to truncate the Taylor expansion of equation (4) at the level of velocity gradients and neglect higher-order derivatives of the velocity field. This approximation has proven effective in describing the chiral drift of helical particles in linear shear flows along the direction normal to the shear plane [4] , [7] . By contrast, we find that chirality-dependent drifting motions in two dimensions require consideration of second-order derivatives of the velocity field along with fourth-order tensors ( ) to describe the detailed shape of the particle. Physically, fluid shear within the Couette cell acts to rotate the particle about its centre as it translates along a circular orbit. The interplay between rotation and orbital translation cause the particle to move back and forth along the radial direction perpendicular to the direction of flow ( Fig. 3c ). Each full rotation of the particle contributes a net displacement that depends on the particle’s chirality as quantified by the chiral factor κ . Although these drifting motions are typically small, their steady accumulation can lead to large displacements over many particle rotations and may, therefore, provide a basis for the hydrodynamic separation of chiral objects. Effects of Brownian motion To assess the possibility of separating smaller micro- and nanoscale objects, we investigate the effect of Brownian motion on the chiral drift velocity through a series of stochastic simulations (see Methods). Briefly, we add a fluctuating force/torque with zero mean and covariance to the otherwise deterministic equations described above. The addition of these Brownian contributions introduces one additional parameter—namely, the thermal energy k B T —which controls the strength of thermal motion relative to the deterministic hydrodynamic motion of the particle. This parameter is conveniently expressed as the inverse of the Péclet number Pe = v c G / D , where v c is the chiral drift velocity in the absence of Brownian motion, D = k B T / K is a characteristic diffusion coefficient ( K =| K | is the magnitude of the resistance tensor K ; for example, K =6 πηa for a sphere of radius a in an unbounded medium) and G is a length scale over which convection and diffusion are compared (for example, the gap width of a Taylor–Couette cell). For each value of the Péclet number, we generate 1,000 stochastic particle trajectories of duration t s =10 T (that is, 10 particle rotations) and calculate the resulting drift velocity, v calc =[ r o ( t s )− r o (0)]/ t s ( Fig. 4 ). For weak thermal agitation ( Pe >>1), the average drift velocity agrees closely with the deterministic result, . By contrast, for strong thermal agitation ( Pe ≪ 1), the particle trajectories are increasingly erratic such that displacement due to chiral drift is increasingly insignificant compared with that of Brownian motion. In the simulations, the length G = v c t s was kept small for computational reasons (simulating the dynamics of microscopic particles over macroscopic lengths was computationally prohibitive); however, the choice of G is arbitrary. Chiral drift (like any convective motion) will ultimately beat out diffusion over large length scales as displacement due to drift scales linearly with time whereas that due to diffusion scales as t 1/2 . In other words, the Péclet number can be made increasingly large by increasing the length G over which the chiral separation is to occur. For a given length G , the separation of particles of opposite chirality should indeed be feasible provided that Pe >>1 such that the effects of Brownian motion are small. 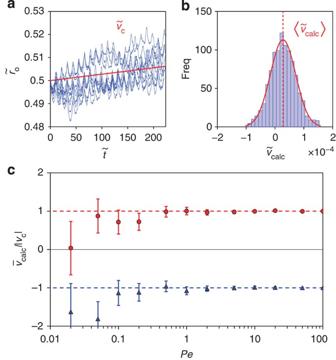Figure 4: Stochastic particles simulations. (a) Ten (of 1,000) stochastic particle trajectories of an R particle (Fig. 3a) for Peclét number,Pe=1. (b) Histogram showing the corresponding distribution of drift velocitiesforPe=1. (c) Average drift velocityas a function ofPefor chiral particles (R and S) shown inFig. 3a; the calculated (calc) drift velocity is scaled by the magnitude of chiral drift |vc| in the absence of Brownian motion. The error bars represent 95% confidence intervals on the mean drift velocity based on 1,000 realizations of the stochastic process. Figure 4: Stochastic particles simulations. ( a ) Ten (of 1,000) stochastic particle trajectories of an R particle ( Fig. 3a ) for Peclét number, Pe =1. ( b ) Histogram showing the corresponding distribution of drift velocities for Pe =1. ( c ) Average drift velocity as a function of Pe for chiral particles (R and S) shown in Fig. 3a ; the calculated (calc) drift velocity is scaled by the magnitude of chiral drift | v c | in the absence of Brownian motion. The error bars represent 95% confidence intervals on the mean drift velocity based on 1,000 realizations of the stochastic process. Full size image Feasibility of chiral separations To separate objects over the gap width G of the Couette cell, transport due to chiral drift must exceed that due to diffusion: v c >> D / G . Approximating the chiral drift velocity as v c ≈ κaL / Tr o and the diffusivity as D ≈ k B T /3 πηL , this condition implies that the particle size must be L >>( k B T / ηω cell ) 1/3 assuming the gap is small (that is, G ≪ R o ). In water ( η =10 −3 Pa˙s) at room temperature ( k B T =4 × 10 −21 J), a Couette cell rotating at a rate of ω cell =10 3 rad s −1 should be capable of separating chiral objects provided L >100 nm. Separating even smaller chiral objects by this mechanism may also be possible in highly viscous fluids—for example, in glycerol ( η =1 Pa˙s), the minimum size is L >10 nm. Interestingly, the chiral drift mechanism described here does not require the alignment of the particle along particular orientations (beyond the initial confinement to the interface) and is, therefore, insensitive to Brownian rotation. The flow-induced rotation of the particle leads—on average—to more rotations in one direction than the other resulting in steady drifting motions. Over sufficiently long times (again corresponding to the condition, Pe >>1), this steady rotational motion will always dominate that of Brownian motion. This behaviour is in sharp contrast with previously reported mechanisms of chiral drift in three dimensions perpendicular to the shear plane [4] , [7] , which require the flow-induced alignment of the particles to achieve steady drifting motions. In these mechanisms, chiral drift vanishes at small scales due to Brownian rotation, which acts to randomize the particle’s orientation. Thus, while the present mechanism is typically weaker than those described previously (for example, v c scales as L 2 as opposed to L ), it may be more robust to Brownian motion at small scales. In summary, we provide conclusive evidence that particles in 2D vortex flows experience in-plane lift forces that depend on particle chirality. This lift force does not vanish at the nanoscale, and should allow for the separation of chiral objects tens of nanometres across even in the presence of Brownian motion. Although the present study focuses exclusively on 2D particles, in-plane lift forces may also act on three-dimensional (3D) chiral objects if and only if they are confined at or near a liquid interface parallel to the shear plane. In the absence of such an interface, rotation of the Couette cell by 180° ( cf. Fig. 2b ) reverses the apparent flow rotation direction but not the chirality of a 3D chiral particle; consequently, in-plane chiral lift forces are prohibited in extended Couette flows by symmetry considerations ( Supplementary Fig. 5 ). To test these predictions, the present experiments should be scaled down and extended to neutrally buoyant particles that can migrate and rotate in 3D; however, the implementation and imaging of such a system is expected to be significantly more challenging. Future models of chirality-selective motions in 3D should incorporate the effects of higher-order velocity gradients ( ∇ ∇ u ) that arise in non-linear flows as these contributions may enable potentially important mechanisms for the hydrodynamic separation of chiral objects. Achiral control experiments Achiral control particles are made using SU-8 photolithography ( Supplementary Fig. 1a ). Both disks (D) and ellipses (E) are made with the same area (in contact with the liquid) and mass as the chiral R and S particles. Experiments are performed in which the direction of rotation of the Couette cell is reversed during the experiment (see dashed vertical line at in Supplementary Fig. 1b ). Upon reversal of the direction, the S particle starts moving towards its steady-state position (see Fig. 2a ), both for the CW to CCW and CCW to CW case ( Supplementary Fig. 1b ). The ellipse E, however, shows a small perturbation in the radial position (due to the sudden reversal of the flow), but quickly returns to the same radial position ( Supplementary Fig. 1b , black and magenta lines). In Supplementary Fig. 1c , we compare the CW versus CCW behaviour of all measured particles (that is, D, E, S and R). No significant differences in angular velocity ω , linear velocity v θ , or radial position r are observed for the achiral particles D and E, whereas R and S chiral particles show significantly different behaviours (as described in the text). These achiral control experiments demonstrate that particle chirality is necessary to obtain changes in ω , v θ and r , when comparing CW versus CCW rotation in Taylor–Couette flows. General hydrodynamic model Equations (2) and (3) describe the motion of a single rigid particle of arbitrary shape moving within an unbounded Stokes flow, u ( r ), in the absence of external forces and torques. To approximate the grand resistance tensor , we first compute the grand mobility tensor though pairwise summation of the far field hydrodynamic interactions between the N spheres that make up the composite particle. This tensor is then inverted to obtain , which includes the long range, many-body interactions between the spheres. Assuming that the distance between neighbouring spheres is large compared with their radius a , the components of the mobility tensor are well approximated as where δ is the identity tensor, η is the fluid viscosity, and r αβ = r β − r α is the vector drawn from sphere α to sphere β. This approach is akin to the Stokesian dynamics method [29] , [30] ; however, it neglects (i) higher-order moments of the force density on the particles’ surface (for example, torques, stresslets, and so on) and (ii) near field (lubrication) interactions between the spheres. Substituting equation (2) for the force on sphere α into the equation (3) for the net force and torque, we obtain where K is the symmetric resistance tensor [25] , Ω is the symmetric rotation tensor [25] , C is the coupling tensor [26] (not necessarily symmetric, C ≠ C † ), and where ε is the alternating unit tensor ( a × b =− a · ε · b ). For the composite particles described here, the resistance tensors are defined explicitly as Equation (6) is directly analogous to that derived by Brenner [28] for the motion of a solid particle and fully specifies the linear and angular velocities of the composite particle. If the particle is small relative to spatial variations in the external flow field, we can approximate the velocity at the position of sphere β by a Taylor series about the particle origin Substituting this approximation into equation (6), we obtain where the tensors n Φ and n Γ are constant n- adic intrinsic resistance coefficients [28] that depend only on the external shape of the particle The level of approximation of equation (9) is precisely that which is required to describe the chiral drift of planar particles in 2D flows ( cf. below). Dynamics of planar particles The dynamical equation (6) is quite general and applies to 3D particles of arbitrary shape moving in any 3D Stokes flow. We now focus our attention on ‘planar’ particles, which are symmetric with respect to reflection about the xy plane, and their movement in 2D flows for which u z =0. In particular, we limit our analysis to unidirectional circular flows of the form as permitted by the incompressible Navier–Stokes equations. The second term is simply rigid body rotation about the origin, which does not contribute to the chiral drift. Without loss of generality, we set c =0. For the Taylor–Couette flow described by equation (1), the first coefficient is . The dynamics of planar particles in this circular flow field is governed by the following system of differential equations (see Supplementary Note 2 for derivation) Here r o and θ o are polar coordinates specifying the position of the particle centre ( Fig. 1b ), γ and φ = γ − θ o are angles specifying the orientation of the particle (relative to the x axis and to the radial vector r o , respectively), and are normalized resistance tensors, and r β is the radial position of sphere β The position specifies the location of sphere β relative to the particle origin using a moving coordinate system, which is fixed to the particle and participates in its motion. Equation (13) governs the dynamics of the position ( r o , θ o ) and orientation ( γ ) of the particle in time. Because these equations depend only on the coordinates r o and φ , we can combine the expressions for and to obtain two differential equations for r o and φ ( cf. below). Equation (13) are integrated numerically using a variable order Adams–Bashforth–Moulton solver with adaptive stepping and a relative error tolerance of 10 −10 to avoid spurious drifting motions. For b >0, particles rotate steadily in the clockwise direction with an angular velocity that depends on their orientation and handedness ( Supplementary Fig. 2b ). The radial position of each particle oscillates in time with a period T equal to that of its rotation and defined by φ ( t + T )= φ ( t )+2 π . Importantly, each rotation contributes a small displacement in the radial direction, and the direction of this steady drifting motion depends on the chirality of the object ( Supplementary Fig. 2c ). Here, R particles move in the positive radial direction; S particles move in the negative radial direction; achiral particles exhibit no such drifting motion. Because the oscillations in the radial direction are small, we can define a local drift velocity v c by averaging the radial velocity over one period of rotation. Numerical evaluation of v c reveals that the magnitude of v c decreases monotonically with distance from the origin as ( Supplementary Fig. 2d ). In the absence of other forces (for example, due to walls of a Taylor–Couette cell), S particles spiral into the origin, and R particles spiral outward indefinitely. In addition, the drift velocity increases quadratically with the size of the chiral particle as v c ∝ L 2 , where L is a characteristic linear dimension of the particle ( Supplementary Fig. 2e ). Below, we develop an analytical approach to approximate v c and confirm the scaling relations observed in the numerical simulations. Scaling analysis To obtain an analytical approximation for the chiral drift velocity, we first expand the governing equations in powers of the object size. Specifically, we modify the size-dependent particle quantities as R α → ε R α and a → εa and expand the governing equation (13) in a power series in ε Here, ε is a dummy value to be set to one at the end of the analysis; the functions f 0 ( φ ), f 1 ( φ ), g 1 ( φ ) and g 1 ( φ ) are given explicitly in Supplementary Note 3 and depend only on components of the tensors characterizing the hydrodynamic shape of the particle. Importantly, the approximation of equations (16) and (17) includes only those terms needed to reproduce the drifting motion of chiral particles (that is, no chiral drift is observed if the series is truncated with fewer terms, and the addition of more terms introduces no new qualitative behaviours). On the basis of this approximation, we now derive analytical estimates for the oscillation period and the chiral drift velocity. At zeroth order in the object size ( ε 0 ), the radial position of the object does not change in time, r o =constant+ O ( ε ); however, the object rotates about its centre as described by where φ ( t )= φ 0 ( t )+ O ( ε ) and the coefficients A and B are constants that depend on the shape of the particle (see Supplementary Note 3 ). Equation (18) implies that the angular velocity oscillates with the particle’s orientation φ reaching a maximum value when the major axis of the object is perpendicular to the streamlines and a minimum value when the major axis is parallel to the streamlines. Such periodic variations in the angular velocity are characteristic of the motion of anisotropic particles in linear shear flows (for example, the Jeffrey orbits [23] of spheroidal particles). Here, the orientation of the particle’s major axis is described by the angle φ m with respect to the X ′ axis where atan2( y , x ) is the four-quadrant inverse tangent function. Equation (18) can then be written as where C 2 = A 2 + B 2 . Integrating this equation over one complete rotation, we obtain the period of rotation, where χ is an effective aspect ratio of the particle defined as This expression for the oscillation period exhibits the same dependence on the particle aspect ratio ( χ ) and the shear rate as the Jeffrey orbits [23] for spheroidal particles in linear shear flows. To approximate the chiral drift velocity and its scaling with particle size, we combine the approximate equations (16) and (17) and expand in powers of the particle size ε to obtain Integrating over one period of oscillation (0≤ φ ≤2 π ), the first term vanishes leaving where Δ r o ≪ r o is the radial displacement after a single particle rotation and K is a chiral factor defined as which depends only on the shape of the particle. The chiral drift velocity v c can now be approximated as the ratio of this displacement and the period of rotation. This is the central result of our analysis. The chiral drift velocity scales with the size of the object as ε 2 and inversely with distance from the origin as in agreement with numerical predictions. Furthermore, the direction and magnitude of the drift velocity depends on the shape of the object as characterized by the chiral factor K . Importantly, the sign of K unambiguously determines the chirality of a 2D object; by arbitrary convention, we assign objects with K <0 as S and K >0 as R. Furthermore, it can be shown that for achiral particles with an additional plane of mirror symmetry, the chiral factor K is identically zero (see Supplementary Note 4 ). Importantly, the chiral drift velocity derived in equation (26) requires the inclusion of hydrodynamic interactions between the spheres that make up the composite particle. In particular, the chiral factor K depends linearly on the sphere radius a as illustrated in Supplementary Fig. 3 . This suggests that the chiral factor scales with the particle size L and the sphere size a as K ~ aL . Therefore, we can defined a dimensionless chiral factor: κ = K / aL , which is at most an order one quantity regardless of particle size; this is the chiral factor that is used in the main text. The dimensionless chiral factor κ depends only on the shape of the particle—for example, the largest drift velocities are achieved for asymmetric particles with large aspect ratios ( Supplementary Fig. 4 ). Effects of Brownian motion To describe the effects of Brownian motion on the dynamics of planar particles moving in rotating flow fields, we start from the Langevin equation for translational and rotational motion, where Here, m is a generalized mass/moment-of-inertia tensor ( m is the mass, I is the moment of inertia), is the particle translational/rotational velocity vector, is the hydrodynamic force/torque vector, and is the stochastic force that gives rise to Brownian motion [29] . At low Reynolds numbers, the hydrodynamic force/torque on the particle is well described by equation (9) or equivalently by equation (4) where The stochastic force/torque arises from thermal fluctuations and is characterized by where k B T is the thermal energy, the angle brackets denote an ensemble average, and δ ( t ) denotes a delta function. The magnitude of the Brownian forces is related to the viscous resistance to motion via the fluctuation-dissipation theorem. The Langevin equation (27) can be integrated [29] in time to give the translational/rotational displacement of the particle in a small time Δ t Here, X B (Δ t ) is a random displacement/rotation due to Brownian motion characterized by The second term of equation (31) represents the deterministic (non-Brownian) component of particle motion as detailed in the previous sections. Importantly, the time step Δ t must be small compared with the time scale of deterministic particle motion (for example, much smaller than the period of the particle’s Jeffrey orbit, Δ t ≪ T ) but also large compared with the Brownian relaxation time τ = m /6 πηL (for example, τ ~10 ps for an L ~10 nm particle in water). Furthermore, when integrating the deterministic contribution of equation (31), care must be taken to avoid numerical errors that can contribute to spurious drifting motions. We use a variable order Adams–Bashforth–Moulton solver with adaptive stepping and a relative error tolerance of 10 −10 in all numerical simulations. The data in Fig. 4 are generated by integrating the stochastic dynamics of a single particle through M rotations (that is, 0≤ φ ≤2 πM ) for different degrees of thermal agitation as characterized by the Peclét number, Pe . The M particle rotations correspond to a characteristic length G = v c TM —the distance over which a particle drifts after M rotations. We used ‘whole’ particle rotations instead of arbitrarily specifying the length G to more accurately estimate the chiral drift velocity as the displacement due to chiral drift can be small compared with variations in the particle’s radial position during a single particle rotation (especially for the relatively short time scales used in the numerical simulations). Such considerations are important even in the absence of Brownian motion. How to cite this article : Hermans, T. M. et al. Vortex flows impart chirality-specific lift forces. Nat. Commun. 6:5640 doi: 10.1038/ncomms6640 (2015).